Origin and elimination of photocurrent hysteresis by fullerene passivation in CH3NH3PbI3planar heterojunction solar cells The large photocurrent hysteresis observed in many organometal trihalide perovskite solar cells has become a major hindrance impairing the ultimate performance and stability of these devices, while its origin was unknown. Here we demonstrate the trap states on the surface and grain boundaries of the perovskite materials to be the origin of photocurrent hysteresis and that the fullerene layers deposited on perovskites can effectively passivate these charge trap states and eliminate the notorious photocurrent hysteresis. Fullerenes deposited on the top of the perovskites reduce the trap density by two orders of magnitude and double the power conversion efficiency of CH 3 NH 3 PbI 3 solar cells. The elucidation of the origin of photocurrent hysteresis and its elimination by trap passivation in perovskite solar cells provides important directions for future enhancements to device efficiency. Organometal trihalide perovskites (OTPs) have recently drawn tremendous research interest as they have demonstrated increased power conversion efficiency (PCE; above 15%) in <5 years of research [1] , [2] , [3] , [4] , [5] , [6] , [7] , [8] , [9] . One of the most attractive features of OTP materials is their ability to form very good polycrystals through low-temperature solution processes [10] , [11] , [12] . Thus, the density of bulk crystal defects in perovskite materials can be much smaller than organic semiconductors in bulk-heterojunction solar cells, contributing to many of their intriguing properties, such as large charge carrier mobility [13] , [14] , long carrier lifetime [14] and recently observed lasing [15] . One big mystery in perovskite solar cell characterization is the presence of large photocurrent hysteresis in many perovskite solar cells, which was recorded by many groups by scanning photocurrents with increasing or decreasing voltages [16] . Generally, a much larger short circuit current density ( J SC ) and open circuit voltage ( V OC ) is recorded if the photocurrent sweep starts from the forward bias (> V OC ) rather than from the reverse bias. Sometimes a fill factor (FF) >100% was observed in our study. Photocurrent hysteresis imposes a serious issue on the accurate determination of perovskite solar cell efficiencies and stability concerns. There are concerns on whether photocurrent hysteresis is an intrinsic property of perovskite materials, which might originate from the possible ferroelectricity of OTPs or the electromigration of ions in OTPs [16] . In this manuscript, we identify the presence of a large density of charge traps as the origin of the notorious photocurrent hysteresis in the planar heterojunction (PHJ) perovskite solar cells, and demonstrate that these traps can be passivated by the fullerene layers deposited on the perovskite layers, which eliminate photocurrent hysteresis and improve device performance. Eliminating photocurrent hysteresis by PCBM passivation The structure of the PHJ devices in this study is indium tin oxide (ITO)/poly(3,4-ethylenedioxythiophene) poly(styrenesulfonate) (PEDOT:PSS)/MAPbI 3 (280 ∼ 320 nm)/Phenyl-C61-butyric acid methyl ester (PCBM) (20 nm)/C 60 (20 nm)/2,9-dimethyl-4,7-diphenyl-1,10-phenanthroline (BCP, 8 nm)/aluminum (Al, 100 nm), as shown in Fig. 1a . The MAPbI 3 layers were formed by a low-temperature solution process, interdiffusion of lead iodide (PbI 2 ) and a methyl ammonium iodide (CH 3 NH 3 I, CH 3 NH 3 =MA) stacking layer followed by a solvent annealing process, which was recently developed in our research group [17] , [18] . It forms smooth, compact perovskite films with 100% surface coverage and gives extremely small low leakage current on the order of 10 −4 ∼ 10 −3 mA cm −2 . The solvent annealing markedly increases the grain size to be comparable to or larger than film thickness, paving the way for the study of the fullerene passivation effect. A cross-section scanning electron microscope (SEM) image is shown in Fig. 2b , revealing the polycrystalline nature of MAPbI 3 . 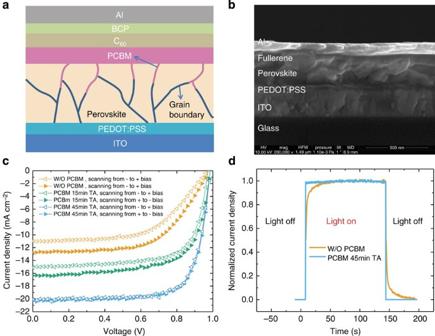Figure 1: Perovskite photovoltaic device structure and performance. (a) Device structure with PCBM layer. (b) Cross-section SEM image of perovskite devices with 45 min thermal annealing (TA) PCBM layer. (c) Photocurrents for devices without a PCBM layer (orange), with PCBM layers thermally annealed for 15 min (green) and 45 min (blue), respectively. Hollow triangles and solid triangles represent the scanning direction from negative to positive bias and from positive to negative bias, respectively. (d) Photocurrent rising process on turning on and turning off the incident light for the devices without PCBM layer (yellow) and with PCBM layer after 45 min thermal annealing (blue). Figure 1: Perovskite photovoltaic device structure and performance. ( a ) Device structure with PCBM layer. ( b ) Cross-section SEM image of perovskite devices with 45 min thermal annealing (TA) PCBM layer. ( c ) Photocurrents for devices without a PCBM layer (orange), with PCBM layers thermally annealed for 15 min (green) and 45 min (blue), respectively. Hollow triangles and solid triangles represent the scanning direction from negative to positive bias and from positive to negative bias, respectively. ( d ) Photocurrent rising process on turning on and turning off the incident light for the devices without PCBM layer (yellow) and with PCBM layer after 45 min thermal annealing (blue). 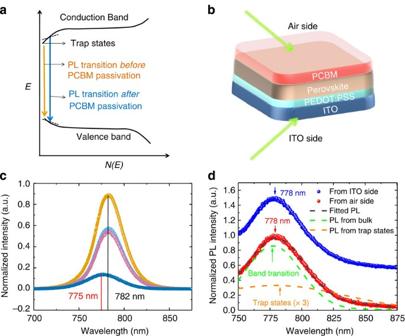Figure 2: Photoluminescence for PCBM passivation effect from different incident directions. (a) Schematic of PL peaks blue-shift from passivation effect. (b) Experiment set-up. (c) The PL spectra for samples with 45 min thermal annealing PCBM layer with 532 nm green laser as excitation source from the air side (dark blue), from the ITO side (pink), and samples W/O PCBM layer from the air side (orange), from the ITO side (sky blue). (d) The PL spectra of the samples with 45 min thermal annealing PCBM layer excited by a 650-nm red laser, with incident light from the air side (red circle line) and from the ITO side (blue circle line, shifted for clarity). The PL spectrum with incident light from the air side were deconvoluted to two peaks, which can be assigned to emission from band transition (green dash line), and from trap states (orange dash line), which was magnified by three times for clarity. Full size image Figure 2: Photoluminescence for PCBM passivation effect from different incident directions. ( a ) Schematic of PL peaks blue-shift from passivation effect. ( b ) Experiment set-up. ( c ) The PL spectra for samples with 45 min thermal annealing PCBM layer with 532 nm green laser as excitation source from the air side (dark blue), from the ITO side (pink), and samples W/O PCBM layer from the air side (orange), from the ITO side (sky blue). ( d ) The PL spectra of the samples with 45 min thermal annealing PCBM layer excited by a 650-nm red laser, with incident light from the air side (red circle line) and from the ITO side (blue circle line, shifted for clarity). The PL spectrum with incident light from the air side were deconvoluted to two peaks, which can be assigned to emission from band transition (green dash line), and from trap states (orange dash line), which was magnified by three times for clarity. Full size image A PCBM/C 60 double fullerene layer was inserted between the perovskite and cathode as an electron acceptor and collection layer [19] , [20] . The PCBM layer was spun onto the perovskite layer followed by low-temperature thermal annealing at 100 °C for varied durations of 0 to 60 min and the C 60 layer was thermal evaporated. We have previously shown that the spun PCBM layer can conformably cover perovskite with intimate contact and permeate into the perovskite layer along the grain boundaries as the thermal annealing proceeds [21] . Controlled devices without PCBM layers were also fabricated with exactly the same parameters except for the PCBM layer. The photocurrents of the control devices show a large hysteresis when scanning the photocurrents with increased or decreased bias at a scan rate of 0.05 V s −1 , as shown in Fig. 1c . Such photocurrent hysteresis is also typically observed in many kinds of electronic devices, particularly defect-rich, organic-based electronic devices, which contain a non-negligible amount of charge traps [22] . The current hysteresis can be explained by the dynamic electric field/charge injection modulated charge trapping and detrapping processes and is intentionally designed for some functional electronic devices, such as bistable memory [23] , [24] . The photocurrent hysteresis decreases with a spun PCBM layer on top of a perovskite layer and completely disappears after annealing the PCBM layer for 45 min. A high PCE of 14.9% under air mass 1.5 global (AM 1.5G) illumination was obtained. Clearly, the application of a PCBM layer with appropriate thermal annealing duration markedly increased the PCE by 204% from 7.3 to 14.9%, which comes mainly from the enhanced J SC and FF. These results demonstrate the presence of a large density of charge traps in annealed MAPbI 3 films, and PCBM can effectively passivate them. This conclusion is also supported by the increased device response speed after passivation. As shown in Fig. 1d , the control devices without PCBM show a slow rising of photocurrent to maximum value during a long duration (75 s) on turning on the illumination, corresponding to the trap filling process, while the photocurrent turns on almost instantly in the optimized devices. The slow rising of photocurrent to maximum also explains J SC calculated from external quantum efficiency curves in many publications. This does not agree with the measured J SC under steady illumination because external quantum efficiency measurement is generally conducted at a much higher lock-in frequency. Origin and the location of the charge traps in MAPbI 3 An important issue that must be addressed is to find out where the traps are in the bulk or at the surface/grain boundaries. Here we used a photoluminescence (PL) study to identify the location of the charge traps by confining the PL light excitation region close to the surface of perovskite layer or through the perovskite films. Generally, the spontaneous radiative recombination between trap states leads to a red-shifted emission peak compared with that from the band edge transition and passivation of these trap states can blue-shift the PL peak, which is illustrated in Fig. 2a . We first used an excitation light of 532 nm, which has a penetration length of 80 nm, much less than the thickness of the perovskite films (280 ∼ 320 nm). The geometry of the PL measurement is shown in Fig. 2b , in which the incident excitation light either from the ITO side or from the air side, and the PL from perovskite films with and without PCBM layers were measured. As shown in Fig. 2c , the perovskite film without a PCBM layer had a PL peak at 782 nm, which is independent of the incident light directions, indicating the top and bottom surfaces have the same optical property. As expected, the perovskite passivated by PCBM had a blue-shifted PL peak from 782 to 775 nm when the top surface was excited, while the PL peak did not show any shift when the incident light came from the ITO side. The results indicate that the PCBM can passivate the trap states close to the top surface and/or along the grain boundaries, and the permeation depth of PCBM in perovskite films after 45 min of thermal annealing should be no more than 200 nm, otherwise the passivation effect should be detected at the ITO side. To verify this hypothesis, a 650 nm continuous red laser, which has a much longer penetration depth comparable to the MAPbI 3 film’s thickness, was used to excite the perovskite films passivated by PCBM. As shown in Fig. 2d , the PL peak shifted to 778 nm, which lies between the 775 and 782 nm, which are assigned to the recombination from the band transition and the trap states, respectively. The PL spectra did not show an obvious shift after changing the incident light directions from the air side to the ITO side. These characterizations can be explained by the fact that the PL emission under red laser excitation comes from the entire film. The PL spectra can be well deconvoluted into two 775 and 782 nm peaks, as shown in Fig. 2d . In addition, a quench of perovskite PL by the PCBM of 70% was also observed, smaller than previously reported results, which may stem from the different thicknesses of the perovskite and PCBM layers and different thermal annealing processes [5] . The PL measurements, with an excitation light of different wavelengths clearly verified that the majority of trap states are close to the surface of the MAPbI 3 films. It can also be inferred that the unpassivated charge traps close to the ITO side have negligible hindrance to the hole collection, and thus the charge traps are most likely electron traps. The presence of a large trap concentration close to the top surface of perovskite thin films can be explained by the low thermal stability of these materials. Compared with the traditional inorganic semiconductors, OTPs are hybrid materials with much lower thermal stability. MAPbI 3 has a reported decomposition temperature of 300 °C (ref. 10 ), but the decomposition at surfaces or grain boundaries may occur at much lower temperatures. A recent study by M. Grätzel group [25] showed that MAPbI 3 decomposed after thermal annealing for a short time at 150 °C, and we found that perovoskites decomposed to PbI 2 at an even lower thermal annealing temperature of 105 °C if the thermal annealing duration was as long as 3 h (ref. 26 ). We infer that the MAPbI 3 film surfaces and grain boundaries should be decomposed at a much shorter thermal annealing time, which yields non-stoichiometry composition and dangling bonds and can cause midgap states and charge traps. As all of the MAPbI 3 films formed by the interdiffusion method used in this study went through thermal annealing of 2 h, it is very likely that these traps originated from the surface decomposition. After establishing that PCBM passivation can eliminate the photocurrent hysteresis in perovskite solar cells, we present evidences of the PCBM passivation effect by direct measurement of trap density before and after passivation, then the electronic transport property change of perovskite films by Hall and transient photocurrent measurements and finally demonstrate the reduced surface charge recombination in devices by impedance spectroscopy (IS) modelling. Thermal admittance spectroscopy (TAS) analysis was used to quantize the reduction of trap states in perovskite films by the passivation of PCBM. TAS is a well-established, effective technique for characterizing both shallow and deep defects, which has been broadly applied in understanding defects in thin film [27] , [28] and organic solar cells [29] . The energetic profile of trap density of states (tDOS) can be derived from the angular frequency dependent capacitance using the equation: [30] where C is the capacitance, ω is the angular frequency, q is the elementary charge, k B is the Boltzmann’s constant and T is the temperature. V bi and W are the built-in potential and depletion width, respectively, which were extracted from the Mott–Schottky analysis. The applied angular frequency ω defines an energetic demarcation, where ω 0 is the attempt-to-escape frequency. The trap states below the energy demarcation can capture or emit charges with the given ω and contribute to the capacitance. As shown in Fig. 3 , there was a relatively large density of defect states on the order of 1 × 10 17 to 1 × 10 19 m −3 in the devices without any fullerene passivation, which explained the large hysteresis of photocurrents observed. The tDOS with an energy level above 0.40 eV (Band 2 and Band 3) decreased by nearly two orders of magnitude just after the spin coating of PCBM on the perovskite films even without thermal annealing. The marked decrease of the tDOS was consistent with the decreased photocurrent hysteresis, indicating the effective passivation of charge traps in perovskite by PCBM. It was noted that the relatively shallow trap states (Band 1, 0.35–0.40 eV) were only slightly passivated by PCBM without thermal annealing. However, after thermal annealing so that the PCBM diffused into perovskite layers along grain boundaries, the density of states in Band 1 reduced significantly, while there was barely any further reduction of deep-trap density. These results indicate that the deep traps located at the surface of the perovskite films can be passivated without thermal annealing, while the shallow traps stay deeper in the perovskite films, such as grain boundaries, which can only be passivated by the diffusion of PCBM into the perovskite layers. 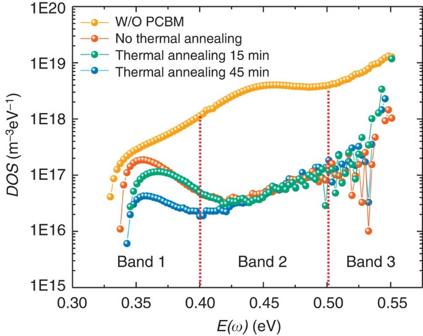Figure 3: Trap density of states (tDOS) obtained by thermal admittance spectroscopy. tDOS for devices without PCBM (orange), with PCBM but no thermal annealing (red), with 15 min thermal annealing PCBM (green), 45 min thermal annealing PCBM (blue). Figure 3: Trap density of states (tDOS) obtained by thermal admittance spectroscopy. tDOS for devices without PCBM (orange), with PCBM but no thermal annealing (red), with 15 min thermal annealing PCBM (green), 45 min thermal annealing PCBM (blue). Full size image To find out the influence of PCBM passivation on the transport properties of the perovskite films, the charge carrier mobility and concentration was investigated using Hall Effect measurements. All of the perovskite films fabricated by the interdiffusion method showed p-type behaviour. It was shown by our previous study that hole mobility was increased from 2.5 to around 30 cm 2 V −1 s −1 after thermal annealing of perovskite films for 1.5 h, saturated with further extended annealing up to 3 h (ref. 26 ). The perovskite films in this study were thermal annealed for 2 h before PCBM deposition, so the mobility change of the perovkite film by thermal annealing can be ignored. 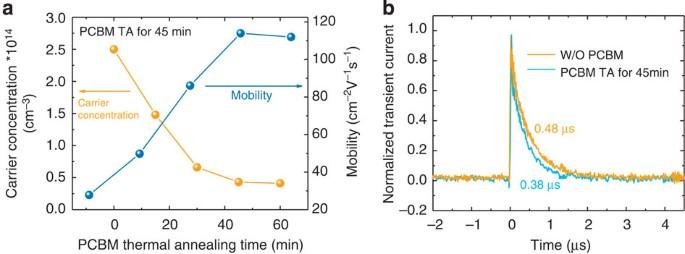Figure 4: Electronic properties of perovskite films without PCBM and with varied PCBM thermal annealing time. (a) Charge carrier concentration (orange) and mobility (blue) by Hall Effect measurements. (b) Charge transient time for samples without PCBM layer (orange) and with 45 min thermal annealing PCBM layer (blue) by transient photocurrent measurement. Figure 4a shows the variation of the carrier concentration and mobility as the duration of PCBM thermal annealing increased, from 15 min to 1 h. Hole mobility continued to increase to 114 cm 2 V −1 s −1 after 45 min of annealing, which is the highest Hall mobility reported [13] . The hole concentration continuously decreased from 2.5 × 10 14 to 4.3 × 10 13 cm −3 as the thermal annealing duration increased from 0 to 45 min. We speculate that the perovskite top surfaces or the grain boundaries tended to decompose on thermal annealing, which introduced more n-doping I vacancies [31] and compensated the p-doping in the original perovskite films. This was confirmed by the reduction in work function with Fermi energy moving closer to midgap on thermal annealing, as observed by a previous ultraviolet photoelectron spectroscopy (UPS) study [26] . After further increasing the thermal annealing time to 60 min, the hole mobility and the carrier concentration became almost invariant. The variation trend of the carrier mobility correlates well with the variation of tDOS: when the tDOS decreases, the hole mobility increases. As Hall effect measurement characterizes the electronic property of the entire film rather than the top surface, it is inferred that PCBM passivates the grain boundaries and reduces the energy barrier between grain domains, facilitating the hole transportation in the plane direction. Figure 4: Electronic properties of perovskite films without PCBM and with varied PCBM thermal annealing time. ( a ) Charge carrier concentration (orange) and mobility (blue) by Hall Effect measurements. ( b ) Charge transient time for samples without PCBM layer (orange) and with 45 min thermal annealing PCBM layer (blue) by transient photocurrent measurement. Full size image The Hall mobility represents carrier transportation behaviour in the plane direction, but, under device operating conditions, the charges transport in the out of plane direction, which means the Hall mobility does not characterize the charge extraction process. To find out how passivation affects the charge collection process, transient photocurrent (TPC) measurement was conducted to measure the average charge transit time across the films after charge generation. As seen in Fig. 4b , the devices with 45 min of thermal annealing a PCBM layer had a shorter charge transient time of 0.38 μs than the devices without a PCBM layer (0.48 μs), corresponding to an enhanced vertical charge carrier transit mobility from 1.9 × 10 −3 to 2.4 × 10 −3 cm 2 V −1 s −1 . We continued to measure the devices under real operating conditions using IS and used modelling to identify the main recombination pathways in OPTs. IS has been widely utilized in many photovoltaic systems, such as dye-sensitized solar cells [32] , organic solar cells [33] and perovskite solar cells [34] , [35] . The technique is a valuable tool to decouple electronic parameters, such as capacitances and resistances in photovoltaic devices, by analysing the frequency-dependent alternating current response with appropriate equivalent circuits. The inset of Fig. 5a shows the equivalent circuit used for our curve fitting, which is similar to that used in organic solar cells by ref. 33 with modification. Here the resistor-capacitor (RC) circuits of the bulk and interface recombination were separated to find out their individual contribution to total charge recombination. The experiment data can be well fitted using this equavelent circuit, as shown in Supplementary Fig. 1 . Two time constants were extracted from the IS modelling, which were assigned to the surface charge recombination with a short charge recombination lifetime (τ surface ) and bulk charge recombination with a much longer charge recombination lifetime (τ bulk ). We assumed that the bulk charge recombination is much slower because the OTP thin films were shown to have excellent crystallinity and low density of bulk defects [15] . τ bulk and τ surface extracted under different bias are shown in Fig. 5a,b . As expected, τ surface is around two orders of magnitude smaller than τ bulk at zero bias and one order of magnitude smaller at V OC , and the overall charge recombination in the devices is dominated by the surface recombination. τ bulk showed little variation under different PCBM passivation conditions, while τ surface increased about three times in whole-bias range after optimizing PCBM annealing conditions, proving our scenario that the PCBM passivation can effectively reduce the surface recombination but have little influence on the bulk recombination. τ bulk is much more sensitive to the applied bias than τ surface , as the bulk charge recombination is sensitive to total injected charge density [14] , while the interface charge recombination is mainly determined by the surface trap density. Therefore, the τ surface increases with the decrease of the surface trap density, matching the tDOS results from the TAS measurements. The IS modelling result demonstrated that surface recombination accounts for the major portion of recombination in the devices, and PCBM passivation can effectively reduce the surface recombination and increase device efficiency. Neverthereless, the τ surface after pasivation is still much smaller than the bulk recombination τ bulk , indicating an opportunity to further improve the device performance with more sophisticated surface passivaiton techniques. 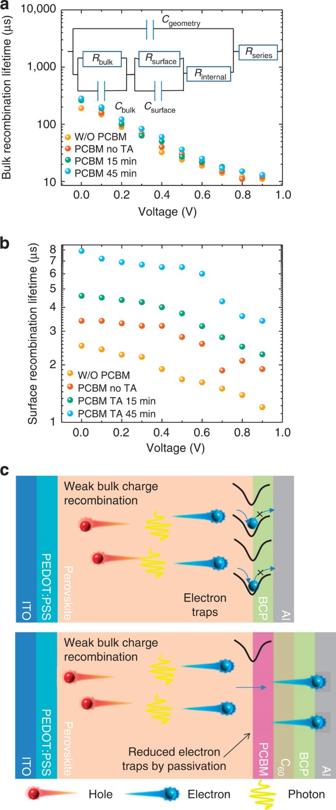Figure 5: Impedance spectroscopy characterization of charge carrier recombination by PCBM passivation. (a) Bulk recombination time and (b) surface recombination time with different PCBM passivation conditions under different applied bias. Inset of (a): the equivalent circuits for impedance spectroscopy fitting. (c) Schematic of the surface recombination reduction by passivating the trap states. Figure 5: Impedance spectroscopy characterization of charge carrier recombination by PCBM passivation. ( a ) Bulk recombination time and ( b ) surface recombination time with different PCBM passivation conditions under different applied bias. Inset of ( a ): the equivalent circuits for impedance spectroscopy fitting. ( c ) Schematic of the surface recombination reduction by passivating the trap states. Full size image The passivation effect of PCBM on the device operation is summarized by the device model shown in Fig. 5c . As the carrier diffusion length in OTP bulk material (721 nm), calculated from τ bulk and transit mobility, is much larger in terms of film thickness, the charges generated in OTPs should be able to reach the surface with negligible loss. The long diffusion length in the bulk of OTP films is reasonable, because the optimized perovskite film thickness is ∼ 600–700 nm while its highest efficiency is 15.6% (ref. 18 ). The electron recombination at the perovskite surface severely reduces the electron extraction efficiency at the cathode side, while PCBM on the perovskite films can effectively passivate these electron traps and markedly reduce the interface charge recombination, which boosts the device J SC and FF. This is further supported by the fivefold smaller series resistance and almost comparable shunt resistance after PCBM passivation, as summarized Supplementary Table 1 . We have revealed and highlighted the importance of the PCBM surface passivation effect to improve perovskite solar cell device performance. The mitigation of defect states is effective, which can be deduced from the significant increase of photocurrent response speed and decrease of the tDOS. Improving electronic properties of perovskite films with optimum fullerene thermal annealing, including a reduced interface charge recombination, a longer charge carrier lifetime and larger mobility, contributed to the very good device performance obtained. It is noted that increasing evidence shows that the working mechanism of perovskite solar cells is similar to other inorganic polycrystalline solar cells such as silicon, cadmium telluride (CdTe) and copper indium gallium selenide (CIGS) solar cells [34] . One of the most important strategies for optimizing device efficiency for all of these polycrystalline solar cells is to minimize the charge recombination at the material surface, electrode interface and grain boundaries by passivating the dangling bonds, which cause a large density of ‘surface states’ in the band gap, as the charge recombination within the crystal grains is negligible when the carrier diffusion length is longer than the crystal grain size. The passivation strategy was proved its merits in the OTP system. Most importantly, our work determined the origin of the photocurrent hysteresis in perovskite solar cells and provides a simple and effective method to eliminate it paving the way for accurate PCE measurements and further efficiency improvements. Film formation and device fabrication PEDOT:PSS (Baytron-P 4083, used as received) was spun on a clean ITO substrate at a speed of 3,000 rounds per minute (r.p.m.). The film was then annealed at 110 °C for 20 min. PbI 2 and MAI were dissolved into dimethylformamide (DMF) and 2-propanol with concentrations of 450 mg ml −1 for PbI 2 and 45 mg ml −1 for MAI, respectively. Both solutions were heated at 100 °C for around 10 min before being used to make sure both MAI and PbI 2 were fully dissolved. The PbI 2 solution was spun on a PEDOT:PSS layer at 6,000 (r.p.m.) for 35 s. Then the PbI 2 film was transferred onto a 70 °C hot plate for quick drying. The MAI solution was then spun on top of dried PbI 2 film at 6,000 r.p.m. for 35 s at room temperature to achieve films with thicknesses ranging from 280–320 nm. The spin-coated PbI 2 /MAI stacking films were annealed at 100 °C for 2 h. After they were cooled down to room temperature, PCBM (dissolved into Dichlorobenzene (DCB), 2 wt %) was spun on top of the formed perovskite layers (for samples with a PCBM layer). After that, the film was annealed at 100 °C for different thermal annealing times to let the PCBM crystalize and diffuse into the perovskite layer. The device was finished by thermal evaporating C 60 (20 nm), BCP (8 nm) and aluminum (100 nm) in sequential order. The device area is the overlap of the ITO substrate and aluminum electrodes (6 mm 2 ). Film and device characterization Simulated AM 1.5G irradiation (100 mW cm −2 ) was produced by a Xenon-lamp-based solar simulator (Oriel 67005, 150 W Solar Simulator) for current-voltage measurement. The light intensity was calibrated by a silicon (Si) diode (Hamamatsu S1133) equipped with a Schott visible-colour glass-filtered (KG5 colour-filtered). The PL spectrum was measured by iHR320 Photoluminescence Spectroscopy at room temperature. A 532-nm green laser with an intensity of 10 mW cm −2 from Laserglow Technologies was used as the excitation source in PL measurement. The thermal admittance spectroscopy was performed using an E4980A Precision LCR Meter from Agilent at frequencies between 0.1 to 1,000 kHz. Hall effect and conductivity measurements were performed with the six contacts van der Pauw method. The contacts were deposited by thermally evaporating 100 nm gold (Au) layers. Indium was used to attach the copper (Cu) wires on the Au contacts. The magnetic field was kept invariant as 0.3 T through the measurements. Keithely 2400 source meter was used to apply DC bias current, and a Keithely 4200 Model was used to record the Hall voltage. All samples were measured in air, under a dark environment, and at room temperature. The validity of the measurement was verified by measuring a standard n-Si sample with 1.8 × 10 14 cm −3 carrier concentration. Impedance spectroscopy was recorded by the E4980A Precision LCR Meter from Agilent with homemade software. For transient photocurrent measurement, 337-nm laser pulses with 4 ns in width and low intensity were applied to the short circuited devices in the dark. The photocurrent produced a transient voltage signal on a 50 Ω resistor, which was recorded by an oscilloscope. Vertical transit mobility calculation The transit mobility μ t is determined by μ t = L 2 / τ t V bi , where L is the thickness of the devices; τ t is the transit time extracted from the transit photocurrent decay curve and V bi is the built-in potential, which is extracted from the Mott–Schottky analysis. How to cite this article: Shao, Y. et al. Origin and elimination of photocurrent hysteresis by fullerene passivation in CH 3 NH 3 PbI 3 planar heterojunction solar cells. Nat. Commun. 5:5784 doi: 10.1038/ncomms6784 (2014).